Fast GCaMPs for improved tracking of neuronal activity The use of genetically encodable calcium indicator proteins to monitor neuronal activity is hampered by slow response times and a narrow Ca 2+ -sensitive range. Here we identify three performance-limiting features of GCaMP3, a popular genetically encodable calcium indicator protein. First, we find that affinity is regulated by the calmodulin domain’s Ca 2+ -chelating residues. Second, we find that off-responses to Ca 2+ are rate-limited by dissociation of the RS20 domain from calmodulin’s hydrophobic pocket. Third, we find that on-responses are limited by fast binding to the N-lobe at high Ca 2+ and by slow binding to the C-lobe at lower Ca 2+ . We develop Fast-GCaMPs, which have up to 20-fold accelerated off-responses and show that they have a 200-fold range of K D , allowing coexpression of multiple variants to span an expanded range of Ca 2+ concentrations. Finally, we show that Fast-GCaMPs track natural song in Drosophila auditory neurons and generate rapid responses in mammalian neurons, supporting the utility of our approach. Imaging of intracellular Ca 2+ has assumed a central role in cellular physiology [1] . Until recently, Ca 2+ has been imaged with small-molecule fluorescent indicator dyes (for example, fura-2 and Oregon Green BAPTA-1), which must be loaded into single cells by pipette or by bulk-loading with low contrast of cell populations. More recently, a promising approach has arisen in the form of genetically encodable calcium indicator proteins (GECIs) [2] , [3] , which are engineered proteins consisting of (i) a Ca 2+ -sensing domain derived from calmodulin or troponin, (ii) a peptide domain that binds the Ca 2+ -sensing domain and (iii) one or more XFP domains whose fluorescence properties are modulated by the Ca 2+ -sensing interaction. GECIs allow cell-type-specific and long-term expression, and have been used to image neuronal circuitry in flies, worms, fish and mammals. Although in recent years the brightness and stability of GECIs have improved, several design challenges remain. First, leading GECIs have slow response kinetics (typically τ on =20 ms—1.4 s and τ off =0.4–5 s) [4] , [5] , [6] , [7] compared with BAPTA-based indicators ( τ on <1 ms and for OGB-1, τ off =7 ms). Physiological Ca 2+ signals can rise within 1 ms and fall in 10–100 ms in small subcellular structures [8] , indicating that slow intramolecular GECI dynamics can limit the ability to resolve spike times and firing rate variations. Second, GECI binding cooperativity is high ( n H =3–4), so that fluorescence signals change over a narrow range of Ca 2+ concentration. For these two reasons, a GECI that can detect single APs is susceptible to saturation during continuous firing; more generally, any given GECI is expected to exhibit most of its brightness change within a proscribed range of firing rates [4] , [6] , [7] . Individual GECIs also do not span the 0.1–10 μM Ca 2+ range over which synaptic plasticity and neurotransmitter release are regulated [9] , [10] , [11] . Here we report the results of a targeted, conservative approach for modifying G reen fluorescent protein/ Ca l m odulin p rotein sensor (GCaMP), a GECI with low degradation, high per-molecule brightness and large fluorescence changes [5] , [7] , [12] . Using GCaMP3 as a starting scaffold, we developed a library of GCaMP variants with a range of affinities and response rates. We found that our variants termed Fast-GCaMPs show faster responses to calcium events in both Drosophila and mammalian neurons. Design principles Our principal goal was to generate accelerated-response GCaMP variants with a variety of affinities. However, we also wished to avoid unintended reductions in maximum brightness ( F max ) and dynamic range ( R f ). We therefore selected target residues for alteration that have not been previously identified to be involved in GFP chromophore stabilization, and either participate in direct Ca 2+ chelation or are at the interface between the calmodulin (CaM) hydrophobic pocket and its binding partner, smooth muscle myosin light-chain kinase peptide RS20 (often incorrectly called M13). CaM contains four EF-hand ‘loop’ domains [13] , each containing up to six residues that form a coordination cage of three acid pairs ( X , Y and Z ; Fig. 1b ). These residues are known to strongly influence binding affinity [14] , [15] , [16] , [17] , [18] . To regulate affinity we designed modifications that increased the number of acidic residues, altered the acid pairings or substituted loop residues with homologous sequences from troponin C [19] ( Fig. 1c , Supplementary Table S1 ). For specific attempts to lower the affinity, we removed one or more acidic chelating residues via Asp→Asn and Glu→Ala substitutions ( Supplementary Table S1 ) [15] , [16] , [18] , [19] . 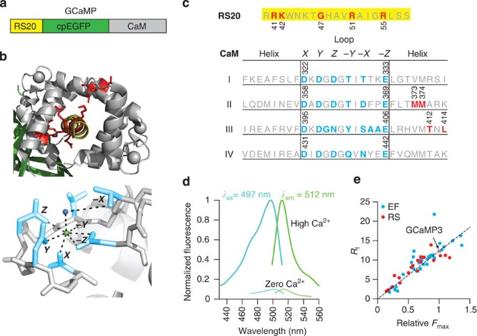Figure 1: Targeted alteration of GCaMP3. (a) GCaMP consists of a cpEGFP fluorophore (green) flanked by an N-terminal RS20 peptide (yellow) and a C-terminal CaM (grey). (b) In the folded state (PDB: 3EVR), RS20 (yellow) and CaM (grey) form an extensive intramolecular interface. Calcium ions are coordinated through six amino acids (red) of the EF-hand loop (blue sphere: water; green sphere: Ca2+ion). (c) Targeted residues in the primary sequence of the RS20 (yellow) and EF-hand (grey) domains with residues at the RS20-CaM interface coloured in blue and residues in the EF-hand loop coloured in red. (d) Mean excitation and emission spectra of Fast GCaMPs. (e) For all 51 variants, dynamic range (Rf=Fmax/Fmin) and maximum brightness (Fmax) relative to GCaMP3 (grey line). Figure 1: Targeted alteration of GCaMP3. ( a ) GCaMP consists of a cpEGFP fluorophore (green) flanked by an N-terminal RS20 peptide (yellow) and a C-terminal CaM (grey). ( b ) In the folded state (PDB: 3EVR), RS20 (yellow) and CaM (grey) form an extensive intramolecular interface. Calcium ions are coordinated through six amino acids (red) of the EF-hand loop (blue sphere: water; green sphere: Ca 2+ ion). ( c ) Targeted residues in the primary sequence of the RS20 (yellow) and EF-hand (grey) domains with residues at the RS20-CaM interface coloured in blue and residues in the EF-hand loop coloured in red. ( d ) Mean excitation and emission spectra of Fast GCaMPs. ( e ) For all 51 variants, dynamic range ( R f = F max / F min ) and maximum brightness ( F max ) relative to GCaMP3 (grey line). Full size image To speed the kinetics of responses to changes in calcium, we targeted internal binding steps. Interaction between GCaMP’s RS20 peptide domain and its CaM domain is required for GCaMP Ca 2+ sensing [20] , [21] . In studies of CaM dynamics, disruptions to the peptide–CaM interaction lead to faster Ca 2+ dissociation [22] . Therefore, we generated point mutations that were likely to disrupt the CaM–RS20 interface [23] , [24] , [25] ( Fig. 1b ). Candidate GCaMP variants span a range of affinities The 51 resulting variants were designated Fast-GCaMP-EF01 through -EF31 (loop variants) and Fast-GCaMP-RS01 through -RS20 (CaM–RS20 interface variants). Variants had the same peak excitation and excitation wavelengths as GCaMP3 ( Fig. 1d ; λ ex =497 nm and λ em =512 nm in n =6 variants tested at high Ca 2+ ), as expected for changes to domains away from the GFP core. To characterize variants in their originally synthesized form we performed Ca 2+ titrations on purified protein to measure R f , Ca 2+ dissociation constant ( K D ) and cooperativity (Hill coefficient or n H ). Of these, 41 had a high/low calcium fluorescence ratio ( R f ) of at least 6. Of those 41 variants, 18 had a maximum, high-calcium brightness ( F max ) of at least 80% of that of GCaMP3 ( Fig. 1e , Supplementary Table S3 ), for a yield rate of 18/51=35%. F max and R f were strongly correlated (Pearson’s correlation r =+0.85), indicating that these parameters were jointly altered by perturbation of the high-fluorescence state. Changes in F max were accompanied by changes in both extinction coefficient and estimated quantum yield ( Table 1 and Supplementary Table 3 ). 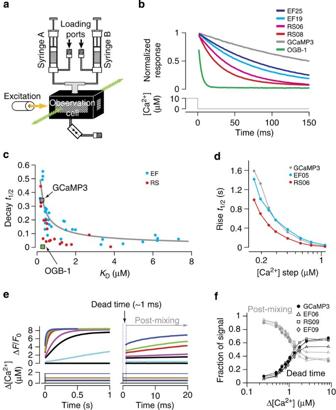Figure 3: Stopped-flow measurement of calcium off- and on-responses from Fast-GCaMPs. (a) Stopped-flow fluorimeter. (b) The fluorescence decay response of selected variants at 37 °C to a step in [Ca2+]freefrom 10 μM to <10 nM. Traces are scaled to the baseline by bi-exponential fit and to the maximum fluorescence intensity at [Ca2+]free=10 μM. (c) Relationship between off-responset1/2andKD(at 25 °C) for variants with mutations at the loop domain (EF variants) or at the RS20–CaM interface (RS variants). The solid line represents a reciprocal curve through the GCaMP3 data point. (d) Calcium-dependence of the rise responses (t1/2) for GCaMP3, EF05, and RS06 at 25 °C. Values smaller than the dead time are plotted as 1 ms. (e) Rise response traces of GCaMP3 to different sizes of [Ca2+] steps from 0. Data are shown at 1-s (left) and 20-ms (right) timescales. The first data point of each ΔF/F0trace represents the magnitude of fluorescence change during the dead time. The magnitude of ΔF/F0during the post-mixing phase is the difference betweenA0(estimated through bi-exponential fitting) and the first recorded point. (f) The magnitude of the signal change during the pre-mixing/dead time (black) and post-mixing (grey) phases as a fraction of the full signal amplitude. One variant (Fast-GCaMP-EF20, K D =6.1 μM) had a 1.37-fold higher F max and a 1.09-fold higher extinction coefficient than GCaMP3. In variants with altered F max , estimated quantum yield tended to change to a greater extent than the extinction coefficient ( Table 1 and Supplementary Table S3 ). Sometimes F min was also affected: one variant (Fast-GCaMP-EF15, K D =1.4 μM) displayed a nearly 1.8-fold increase in R f through a reduction in baseline brightness ( Fig. 2a , Supplementary Table S3 ). 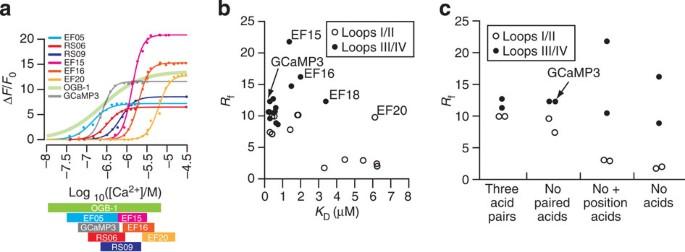Table 1 Biophysical properties of selected novel GCaMP3 variants. Figure 2: Equilibrium fluorescence properties of purified GCaMP3 variants. (a) Ca2+titration of GCaMP3, OGB-1 and six novel GECIs. Solid curves represent fits to the Hill equation. Horizontal bars represent the Ca2+-sensitive range (5–95% of total fluorescence change). (b) Dynamic range as a function ofKD. Each data point represents one variant. Open circles: N-lobe variants. Closed circles: C-lobe variants. (c) The dependence of the dynamic range on the combination of loop acidic residues and the EF-hand site. Three acid pairs: all residues at chelating positions are acidic residues. No paired acids: one/two acidic residues are removed to eliminate acid pairs. No+position acids: acidic residues at +X/+Y/+Zpositions are neutralized to N/N/N (N: Asparagine). No acids: all Asp and Glu are replaced with Asn and Ala, respectively. Full size table Figure 2: Equilibrium fluorescence properties of purified GCaMP3 variants. ( a ) Ca 2+ titration of GCaMP3, OGB-1 and six novel GECIs. Solid curves represent fits to the Hill equation. Horizontal bars represent the Ca 2+ -sensitive range (5–95% of total fluorescence change). ( b ) Dynamic range as a function of K D . Each data point represents one variant. Open circles: N-lobe variants. Closed circles: C-lobe variants. ( c ) The dependence of the dynamic range on the combination of loop acidic residues and the EF-hand site. Three acid pairs: all residues at chelating positions are acidic residues. No paired acids: one/two acidic residues are removed to eliminate acid pairs. No+position acids: acidic residues at + X /+ Y /+ Z positions are neutralized to N/N/N (N: Asparagine). No acids: all Asp and Glu are replaced with Asn and Ala, respectively. Full size image Although full acidification of the X – Z pairs in synthetic loop III peptides has been reported to increase affinity [26] , in GCaMP3 this change did not reduce K D (Fast-GCaMP-EF04, Supplementary Table S3 ). Similarly, acidification of Y – Z pairs [18] did not increase affinity when applied to loop II (Fast-GCaMP-EF02), loop IV (Fast-GCaMP-EF03) or loops I and II (Fast-GCaMP-EF01, Supplementary Table S3 ). Next we altered non-chelating residues by recombining fragments of troponin C (TnC) with the GCaMP3 CaM domain. In previous CaM–TnC chimeras, replacements within the C-lobe (loops III and IV) increased affinity [19] , [27] and accelerated off-binding [19] . To avoid interfering with RS20 interactions, we avoided modifying the CaM helix domains and only substituted up to six TnC residues in loop III (Fast-GCaMP-EF05, residues 397-399; Fast-GCaMP-EF06, residues 397-399 and 403-405, Fig. 1c , Supplementary Table S1 ). Fast-GCaMP-EF06 was unchanged in affinity, but Fast-GCaMP-EF05 showed a 1.6-fold improvement ( K D =155±7 nM, 95% CI, Supplementary Table S3 ) and reduced cooperativity ( n H =2.0±0.3, 95% CI). Among all loop mutants, K D values spanned a range from 0.16 to 6 μM ( Fig. 2a ), permitting the monitoring of a wide range of [Ca 2+ ] free . Mutation of X - and Z -pairs has previously been shown to influence magnesium affinity [15] . In Fast-GCaMP-EF05, -EF20 and -RS06 variants, an IC 50,Mg of 0.3–40 mM Mg 2+ was needed to reduce fluorescence by 50%. The ratio IC 50,Mg / K D,Ca was 2,000–6,000, comparable to values of 2,000–4,000 for GCaMP3 and GCaMP5G. Thus, in our variants the calmodulin domain’s ionic selectivity remained intact. The N-lobe is needed for a functional probe To further explore the participation of acid pairs in binding and fluorescence change, we modified one loop at a time by progressively more disruptive changes: (1) introducing three acid pairs (substitution with Asp); (2) creating half-pairs by neutralizing acidic residues; (3) neutralizing+position residues and (4) neutralizing all acidic residues ( Fig. 2c , Supplementary Tables S1 and S3 ). We found that all changes increased K D , while R f decreased only with disruptions to the N-lobe ( Fig. 2c , Supplementary Table S3 ). When all acidic residues were neutralized, the average R f of the N-lobe mutants was 1.9±0.2 (mean±s.d. ), compared with 12.6±5.2 for C-lobe mutants ( Supplementary Table S3 ). In addition, at the N-lobe variant with highest K D (6.1 μM, EF20), R f was reduced. In summary, strong calcium binding to loops I and II in combination was necessary to give a functional GECI. Disruption of CaM–RS20 interactions accelerates kinetics To characterize response kinetics, we used stopped-flow fluorometry with ~1 ms steps in Ca 2+ concentration ( Fig. 3a ). For a step down in free [Ca 2+ ] from 10 μM to zero (<10 nM) ( Fig. 3b ), most variants responded with a double exponential time course ( Supplementary Tables S4 and S5 ). We measured the decay half-life ( t 1/2 ), as 150 ms (37 °C) and 344 ms (25 °C) for GCaMP3 and 5 ms (37 °C) for Oregon Green BAPTA-1 (OGB-1). Decay responses of GCaMP5 variants [7] are comparable with those of GCaMP3 ( Supplementary Fig. S2A, D ). Figure 3: Stopped-flow measurement of calcium off- and on-responses from Fast-GCaMPs. ( a ) Stopped-flow fluorimeter. ( b ) The fluorescence decay response of selected variants at 37 °C to a step in [Ca 2+ ] free from 10 μM to <10 nM. Traces are scaled to the baseline by bi-exponential fit and to the maximum fluorescence intensity at [Ca 2+ ] free =10 μM. ( c ) Relationship between off-response t 1/2 and K D (at 25 °C) for variants with mutations at the loop domain (EF variants) or at the RS20–CaM interface (RS variants). The solid line represents a reciprocal curve through the GCaMP3 data point. ( d ) Calcium-dependence of the rise responses ( t 1/2 ) for GCaMP3, EF05, and RS06 at 25 °C. Values smaller than the dead time are plotted as 1 ms. ( e ) Rise response traces of GCaMP3 to different sizes of [Ca 2+ ] steps from 0. Data are shown at 1-s (left) and 20-ms (right) timescales. The first data point of each Δ F / F 0 trace represents the magnitude of fluorescence change during the dead time. The magnitude of Δ F / F 0 during the post-mixing phase is the difference between A 0 (estimated through bi-exponential fitting) and the first recorded point. ( f ) The magnitude of the signal change during the pre-mixing/dead time (black) and post-mixing (grey) phases as a fraction of the full signal amplitude. Full size image For Fast-GCaMP-EF variants and GCaMP3 itself, we observed an approximately reciprocal relationship between K D and t 1/2,decay (25 °C, Fig. 3c , curve), reminiscent of the close relationship between affinity and off-binding observed for BAPTA-based indicators [28] . These responses were comparable to those of GCaMP3 and GCaMP5 variants ( Supplementary Fig. S2A ). However, Fast-GCaMP-RS variants did not follow this relationship ( Fig. 3c ), instead showing decay responses up to 6.5-fold faster ( Fig. 3b ) than EF variants of a comparable K D (for decay t 1/2 values measured at 37 °C see Supplementary Fig. S1 and Supplementary Table S5 ). Mutations at the CaM surface of the interface (M373Q, RS05 and M374Q, RS06, Fig. 3c , Supplementary Table S2 ) accelerated off-responses by 5.5- and 4.4-fold, respectively, without significant loss of affinity or R f . In the RS20 domain, the L414T mutation (Fast-GCaMP-RS08 and Fast-GCaMP-RS09, Fig. 3c , Supplementary Table S2 ) accelerated the decay response while increasing K D by 2.5-fold. Rise times were also accelerated in RS mutations. The rise t 1/2 decreased with increasing Δ[Ca 2+ ] ( Fig. 3d ). In comparison to GCaMP3, RS06 showed a 60% increase in rise rate at Δ[Ca 2+ ]=100 nM and a 100% increase at Δ[Ca 2+ ]=570 nM, indicating faster on-responses at physiological concentrations. No improvements in rise responses were detected in GCaMP5 variants [7] ( Supplementary Fig. S2B,C ). For calcium concentrations above (and sometimes below) 2 μM, on-responses were faster than the dead time (~1 ms) of the instrument ( Fig. 3e ). In summary, hydrophobic residues at the CaM–RS20 interface are rate-limiting in both on- and off-responses. For monitoring in vivo Ca 2+ transients we selected RS05, RS06, RS08 and RS09 ( Table 1 ). Several features of the on-responses indicated the presence of a combination of fast and slow processes ( Fig. 3e ): first, rise responses at all values of Δ[Ca 2+ ] had at least two exponential components; second, rise kinetics were not saturated at concentrations for which equilibrium fluorescence was near-maximal and third, the first data point after the mixing dead time (~1 ms) was increasingly elevated from baseline with increasing values of Δ[Ca 2+ ]. For example, for GCaMP3, within the dead time the fluorescence change was 10% complete at Δ[Ca 2+ ]= K D =250 nM, 50% at Δ[Ca 2+ ]=1 μM and 65% at Δ[Ca 2+ ]=10 μM ( Fig. 3f ). Similar observations were made for all tested variants, with half-maximal amplitudes of the pre-dead-time phase appearing at concentrations of >1 μM. These observations are consistent with the existence of a rapid low-affinity binding step that can drive transition to a high-fluorescence state. Imaging sensory-evoked Ca 2+ activity in Drosophila As our first test of in vivo performance, we expressed variants in Drosophila melanogaster ( Fig. 4a ) and optically monitored responses to sound stimuli along the antennal nerve, in a subset of mechanosensory neurons (Johnston’s organ neurons, JONs; Fig. 4a ). JON population activity as assessed by field potential recording is highly reproducible between stimulus trials [29] . We analyzed small regions of interest (ROIs) comprising ~5 axons per ROI. We used two types of song stimuli: a 10-s natural courtship song, containing both sine and pulse song ( Fig, 4c ), and synthetic song pulse trains ( Fig. 4h ). 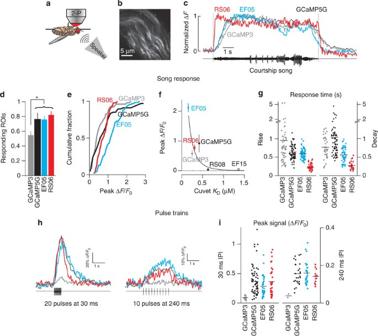Figure 4: Responses of Fast-GCaMPs inDrosophila. (a) Two-photon imaging of responses to sound inDrosophilaantennal nerve. (b) Expression of the EF05 variant in antennal nerve axons 2 days after eclose (scale bar, 5 μM). (c) Normalized example responses toD. melanogastercourtship song. Full scale corresponds to a ΔF/F0range of GCaMP3 70%, GCaMP5G 60%, EF05 100%, and RS06 50%. (d) Fraction of responding ROIs (‘*’ representsP<0.005 by Fisher’s exact test, GCaMP3,n=95 ROIs, four animals; GCaMP5G,n=92 ROIs, seven animals; EF05,n=83 ROIs, three animals; RS06,n=56 ROIs, 3 animals; error bars, s.e.m.). (e) Cumulative distribution of peak fluorescence amplitudes (peak ΔF/F0). (f) Peak ΔF/F0. The dependence of peak ΔF/F0onKD(black line) is calculated usingnH=3 (error bar: s.e.m.; RS08: filled black circle; EF15: open black circle). (g) Rise (left) and decay (right) times (t1/2) of song-responsive ROIs for GCaMP3 (rise,n=53 ROIs; decayn=39 ROIs), GCaMP5G (rise,n=72 ROIs; decay,n=69 ROIs), EF05 (rise,n=63 ROIs; decay,n=54 ROIs) and RS06 (rise,n=46 ROIs; decay,n=34 ROIs). (h) Example fluorescence responses to trains of sound pulses (black). (i) Responses (ΔF/F0) to sound pulses at 33 Hz (left, 30 ms IPI) and 4.2 Hz (right, 240 ms IPI). Line segments represent means. GCaMP3 (grey), GCaMP5G (black), EF05 (cyan) and RS06 (red). Figure 4: Responses of Fast-GCaMPs in Drosophila. ( a ) Two-photon imaging of responses to sound in Drosophila antennal nerve. ( b ) Expression of the EF05 variant in antennal nerve axons 2 days after eclose (scale bar, 5 μM). ( c ) Normalized example responses to D. melanogaster courtship song. Full scale corresponds to a Δ F / F 0 range of GCaMP3 70%, GCaMP5G 60%, EF05 100%, and RS06 50%. ( d ) Fraction of responding ROIs (‘*’ represents P <0.005 by Fisher’s exact test, GCaMP3, n =95 ROIs, four animals; GCaMP5G, n =92 ROIs, seven animals; EF05, n =83 ROIs, three animals; RS06, n =56 ROIs, 3 animals; error bars, s.e.m.). ( e ) Cumulative distribution of peak fluorescence amplitudes (peak Δ F / F 0 ). ( f ) Peak Δ F / F 0 . The dependence of peak Δ F / F 0 on K D (black line) is calculated using n H =3 (error bar: s.e.m. ; RS08: filled black circle; EF15: open black circle). ( g ) Rise (left) and decay (right) times ( t 1/2 ) of song-responsive ROIs for GCaMP3 (rise, n =53 ROIs; decay n =39 ROIs), GCaMP5G (rise, n =72 ROIs; decay, n =69 ROIs), EF05 (rise, n =63 ROIs; decay, n =54 ROIs) and RS06 (rise, n =46 ROIs; decay, n =34 ROIs). ( h ) Example fluorescence responses to trains of sound pulses (black). ( i ) Responses (Δ F / F 0 ) to sound pulses at 33 Hz (left, 30 ms IPI) and 4.2 Hz (right, 240 ms IPI). Line segments represent means. GCaMP3 (grey), GCaMP5G (black), EF05 (cyan) and RS06 (red). Full size image We expected that on average, higher-affinity variants would generate larger signals to the same courtship song. For Fast-GCaMP-EF05 and another high-affinity variant, Fast-GCaMP-RS06 ( Fig. 4d ), more ROIs showed measurable responses than GCaMP3 and the overall distribution of responses was shifted to larger values of peak Δ F / F 0 ( Fig. 4e ; Fast-GCaMP-RS06, P =0.0025; Fast-GCaMP-EF05, P <10 −6 , Kolmogorov–Smirnov test). Low-affinity variants (Fast-GCaMP-RS09, -EF15 and -EF18) generated little to no fluorescence increase, whereas the highest-affinity variant (Fast-GCaMP-EF05) outperformed GCaMP3 by 3.7-fold ( Fig. 4f ) and GCaMP5G by 2.4-fold. In summary, Fast-GCaMP variants retained their calcium-sensitive reporting properties in the form of increased fluorescence change. To test the song response speeds for two variants (Fast-GCaMP-EF05 and Fast-GCaMP-RS06), we estimated the rising and falling t 1/2 in ROIs with a response signal-to-noise ratio (SNR) of at least 2. Compared to GCaMP3 and GCaMP5G, Fast-GCaMP-RS06 performed 3–4 times faster, whereas Fast-GCaMP-EF05 performed only 1.4–1.6-fold faster ( Table 2 and Fig. 4g ). Rise and decay times for the new variants tended to be less variable (Fast-GCaMP-RS06: CV rise =0.36, CV decay =0.40; Fast-GCaMP-EF05: CV rise =0.23, CV decay =0.35) than for GCaMP3 (CV rise =1.02, CV decay =0.45) and GCaMP5G (CV rise =0.31, CV decay =0.68). Table 2 In vivo response times of Fast-GCaMPs. Full size table We also tested responses to trains of 10 song pulses with 240 ms interpulse intervals (IPI) and 20 song pulses with 120, 60 and 30 ms IPI ( Fig. 4h ). In ROIs that responded (SNR>2) to low frequency stimulation (10 pulses at 240 ms IPI), the peak Δ F / F 0 was 3.8±1.3% for GCaMP3 (mean±s.d., n =2 responding out of 45 ROIs), whereas the peak of Fast-GCaMP-EF05 and Fast-GCaMP-RS06 responses were 15.9±6.0% ( n =28 responding out of 35 ROIs) and 14.0±3.7% ( n =12 responding out of 34 ROIs) respectively, comparable to GCaMP5G (15.4±5.8%, n =27 responding out of 92 ROIs; Fig. 4i ). Such a performance improvement over GCaMP3 for stimuli spaced at 240 ms is consistent with the high affinity and the faster response of the two Fast-GCaMP variants. Responses to short, high-frequency pulses (20 pulses at 30 ms IPI) were also larger for the new variants and GCaMP5G (Fast-GCaMP-EF05, 35±16%; Fast-GCaMP-RS06, 39±22%; and GCaMP5G, 37±24% versus GCaMP3, 11±5%; mean±s.d. ; Fig. 4i ), with Fast-GCaMP-RS06 showing an average off-response time of t 1/2 =0.25±0.01 s ( Supplementary Figure S3 ). Lastly, we measured responses to single synthetic pulses and found that none of the GECIs tested generated measurable signals. Thus, high affinity (Fast-GCaMP-EF05) and fast response (Fast-GCaMP-RS06) were associated with improved responses to both natural song and synthetic song pulse trains. Characterization of Fast-GCaMPs in mammalian neurons As our second in vivo functional test, we used two preparations to assess performance in mammalian neurons ( Fig. 5a and Table 2 ). Rat superior cervical ganglion neurons (SCGN) were cultured for 9–14 days before infection with the common neuroanatomical tracing strain pseudorabies virus (PRV) Bartha-expressing GCaMP3 or Fast-GCaMP-EF05, -RS05 or -RS09. Responses to extracellular stimulation were imaged from axonal protrusions using two-photon microscopy in line scan mode (2 ms per line). Mouse layer 2/3 (L2/3) pyramidal neurons were imaged in brain slices from 14–21-day-old mice following embryonic in utero electroporation of GCaMP3, GCaMP5G or Fast-GCaMP-EF05, -RS06 or -EF13. Action potentials were evoked by current injection in whole-cell patch recordings (typical responses, Fig. 5b ). 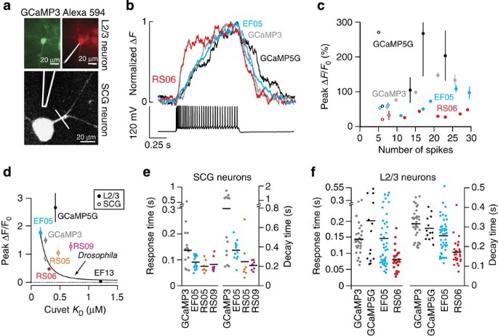Figure 5: Responses of fast GCaMPs in superior cervical ganglion and neocortical pyramidal neurons. (a) Top left: Epifluorescence image of layer 2/3 pyramidal neuron expressing GCaMP3 in acute brain slice form postnatal day 16 mouse. Top right: Same cell filled with Alexa Fluor 594 hydrazide by whole-cell patch electrode (depicted by drawing). Bottom: two-photon image of cultured mouse SCGN expressing GCaMP3 8 h post-infection. The white line represents the axonal scan location. The outline depicts the location of the stimulation electrode. (b) Normalized example traces of fluorescence responses to action potentials elicited by a depolarizing current step in layer 2/3 pyramidal neurons at 35 °C when monitored with GCaMP3 (grey), GCaMP5G (black), EF05 (cyan), and RS06 (red). Full scale corresponds to a ΔF/F0range of GCaMP3 120%, GCaMP5G 500%, EF05 120% and RS06 50%. (c) In layer 2/3 pyramidal neurons, the peak ΔF/F0was correlated with the number (4 or greater) of evoked spikes. Peak ΔF/F0is the mean of three-spike bins and error bars represent s.e.m.. Open circles: 100 ms depolarization step; closed circles: 1 s depolarization step. (d) Relationship between peak ΔF/F0and the affinity of the variant for both SCGN (open circles) and layer 2/3 pyramidal neurons (closed circles; for SCGN: GCaMP3,n=7; EF05,n=10; RS05,n=7, RS09,n=5; for L2/3: GCaMP3,n=3; GCaMP5G,n=5; EF05,n=7; RS06,n=5). Error bars, s.e.m. (e) Kinetics of Ca2+-mediated fluorescence responses. SCGN processes for GCaMP3 (grey), EF05 (cyan), RS05 (orange) and RS09 (pink). (f) Layer 2/3 pyramidal neurons for GCaMP3 (grey), GCaMP5G (black), EF05 (cyan), RS06 (red). Line segments indicate means. Figure 5: Responses of fast GCaMPs in superior cervical ganglion and neocortical pyramidal neurons. ( a ) Top left: Epifluorescence image of layer 2/3 pyramidal neuron expressing GCaMP3 in acute brain slice form postnatal day 16 mouse. Top right: Same cell filled with Alexa Fluor 594 hydrazide by whole-cell patch electrode (depicted by drawing). Bottom: two-photon image of cultured mouse SCGN expressing GCaMP3 8 h post-infection. The white line represents the axonal scan location. The outline depicts the location of the stimulation electrode. ( b ) Normalized example traces of fluorescence responses to action potentials elicited by a depolarizing current step in layer 2/3 pyramidal neurons at 35 °C when monitored with GCaMP3 (grey), GCaMP5G (black), EF05 (cyan), and RS06 (red). Full scale corresponds to a Δ F / F 0 range of GCaMP3 120%, GCaMP5G 500%, EF05 120% and RS06 50%. ( c ) In layer 2/3 pyramidal neurons, the peak Δ F / F 0 was correlated with the number (4 or greater) of evoked spikes. Peak Δ F / F 0 is the mean of three-spike bins and error bars represent s.e.m.. Open circles: 100 ms depolarization step; closed circles: 1 s depolarization step. ( d ) Relationship between peak Δ F / F 0 and the affinity of the variant for both SCGN (open circles) and layer 2/3 pyramidal neurons (closed circles; for SCGN: GCaMP3, n =7; EF05, n =10; RS05, n =7, RS09, n =5; for L2/3: GCaMP3, n =3; GCaMP5G, n =5; EF05, n =7; RS06, n =5). Error bars, s.e.m. ( e ) Kinetics of Ca 2+ -mediated fluorescence responses. SCGN processes for GCaMP3 (grey), EF05 (cyan), RS05 (orange) and RS09 (pink). ( f ) Layer 2/3 pyramidal neurons for GCaMP3 (grey), GCaMP5G (black), EF05 (cyan), RS06 (red). Line segments indicate means. Full size image In mammalian neurons, peak Δ F / F 0 scaled inversely with in vitro K D ( Fig. 5d ), with the largest responses for the highest-affinity variant (Fast-GCaMP-EF05, n =10 SCGN and n =7 L2/3 pyramidal neurons) and no detectable response for the EF13 variant ( n =6 neurons), similar to performance in Drosophila ( Fig. 5d , curve). The peak Δ F / F 0 for GCaMP5G ( n =5 neurons) was variable but on average greater than both GCaMP3 and Fast-GCaMP variants. In L2/3 neurons expressing GCaMP3, GCaMP5G, Fast-GCaMP-EF05 and Fast-GCaMP-RS06, we observed a strong correlation between number of evoked action potentials and peak fluorescence ( Fig. 5c ). To quantify response times in both SCGN ( Fig. 5e ) and L2/3 neurons ( Fig. 5f ), we estimated time to first response ( t response ) and decay t 1/2 ( Table 2 ). We calculated t response as the time to reach an SNR of >2. In SCG neurons, Fast-GCaMP-EF05, -RS05 and -RS09 all had response and decay times shorter than GCaMP3 and GCaMP5G. In L2/3 neurons, Fast-GCaMP-RS06 and Fast-GCaMP-EF05 also had shorter response/decay times than GCaMP3 and GCaMP5G, with the exception of the EF05 response time. Taken together, our results show that the increased sensitivity and speed of Fast-GCaMP-EF and Fast-GCaMP-RS variants are associated with improved reporting performance when expressed in situ . By making targeted changes in Ca 2+ -sensing components of GCaMP3, we have generated a series of variants termed Fast-GCaMPs. Fast GCaMPs respond to Ca 2+ with up to 20-fold improved kinetics and have affinities spanning the range of intracellular neuronal Ca 2+ signals while retaining their per-molecule brightness. Recent research leading to improved GCaMP variants involved screening thousands of mutants generated by exhaustive mutagenesis to yield improvements in proteolytic stability and per-molecule fluorescence [5] , [7] . Another effort has led to similar brightness improvements and modest kinetic improvements [7] . Although a combinatorial approach can be effective at maximizing one parameter at a time, parameters such as K D , decay response and rise response present a challenge because they are often linked to one another. Our results demonstrate that functional parameters of a GECI can be engineered without losing existing beneficial features, and can lead to kinetic improvements beyond previous fast-responding GECIs including TN-XL and GCaMP1.6 (decay τ =240–260 ms) [30] , [31] . For kinetic optimization, our quantitative evaluation of Fast-GCaMP variants required an evaluation method in which cellular calcium dynamics are not a rate-limiting factor. The time course of cellular fluorescence signals is limited by both calcium dynamics and probe response kinetics. As an illustration of why these factors matter, a recent GCaMP optimization effort [12] showed an improvement in physiological off-responses from t 1/2 =0.6 s using GCaMP3 to t 1/2 =0.4 s using their variants of GCaMP6 and GCaMP8. However, those measurements were done in slice cultures in which calcium removal mechanisms were slower than in acute slices, as evidenced by the slow GCaMP3 responses. Our fastest physiological off-response times were several times faster, t 1/2 =0.1–0.2 s for RS06 and RS09, and we found that stopped-flow measurements on purified protein were faster still, with t 1/2 =7–30 ms. In addition, the variant of GCaMP6 produced by Ohkura et al . [12] and GCaMP8 did not have shorter rising t 1/2 than GCaMP3, whereas our Fast GCaMPs showed faster-rising responses than GCaMP3, both in Drosophila and in neocortical L2/3 neurons. Although these measurements all point toward our variants having the fastest responses, direct comparison of GCaMP kinetic performance will ultimately require either stopped-flow measurements or an expression system in which calcium signals are extremely rapid (for example, single spikes in unbuffered dendritic spines [8] ). Our finding of a submillisecond response for calcium steps > K D is consistent with previous observations on GCaMP1.6 (ref. 32 ) and calmodulin itself [33] . GCaMP may therefore have a low-affinity binding state capable of rapid transition to a high-fluorescence state. A likely rapid-binding candidate is the low-affinity pair of sites at the N-domain [33] , an idea that is consistent with our observation that chelation by N-domain loops I and II is necessary to generate a functional probe. A second target for perturbation was the interaction between CaM and its target. Upon Ca 2+ binding, CaM must interact with RS20 to allow a conformational change to a high-fluorescence state. Ca 2+ dissociation from the high-fluorescence state is energetically unfavored because RS20 binding increases Ca 2+ affinity [22] . Consistent with this concept is the recent observation that alterations in a linker domain led to both strongly increased affinity and considerable slowing of off-responses, indicating that bound Ca 2+ is effectively trapped [6] . The relatively bright GECI YC-Nano15 has high affinity, making it useful for detecting single action potentials [34] ; however, high affinity is accompanied by extremely slow off-kinetics, precluding the tracking of successive spikes occurring at high frequency. The same difficulty is apparent for the faster GCaMP5 family of GECIs [7] . Our findings demonstrate the converse point: perturbations to CaM—RS20 interactions decreased affinity and led to considerable speeding of off-responses. We constructed a molecular dynamics model based on our observations. Several conditions had to be satisfied: (1) based on our results, the elimination of Ca 2+ binding in any EF-hand loop resulted in reduced Ca 2+ affinity, indicating cooperative interactions among the four EF-hand sites ( Supplementary Tables S2 and S3 ). (2) Deletion of residues from the RS20 peptide can severely disrupt probe activity ( Supplementary Tables S2 and S3 ), indicating a necessary role for RS20 in reaching both high fluorescence and high Ca 2+ affinity. (3) Elimination of either loop I or loop II leads to a significant reduction in R f ( Fig. 2c ), indicating a necessity for Ca 2+ binding to both sites of the N-lobe to achieve protection of the chromophore and conformational changes that lead to high fluorescence. (4) The elimination of Ca 2+ binding to loop III or loop IV led to reduced Ca 2+ affinity and left the R f intact ( Fig. 2b ), indicating that the C-lobe is required for high-affinity Ca 2+ binding but not for chromophore protection. (5) Based on our discovery of the fast, submillisecond rise response and experimental evidence described by Faas et al . [33] , binding of Ca 2+ to the N-lobe occurs on a submillisecond timescale, with lower affinity than the slower-binding C-lobe ( Figs 4a and 5b ). We propose a kinetic model in which GCaMP has two pathways to a high-fluorescence state ( Fig. 6 ). Loops I and II (N-lobe) begin in a low-affinity (1 μM) state, while loops III and IV (C-lobe) begin in a high-affinity (250 nM) state. In ‘C-like’ activation for small Ca 2+ transients, Ca 2+ would bind to the C-lobe with slow kinetics. The bound C-lobe then acts via interactions with the RS20 domain to increase the calcium affinity of the N-lobe [22] . After the N-lobe binds to Ca 2+ , the entire CaM–RS20 complex shifts in conformation [20] , leading to reduced chromophore-solvent access, leading to a high-fluorescence state. 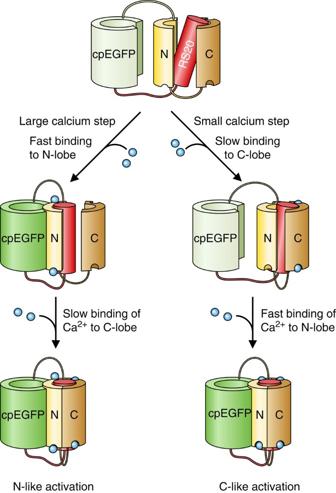Figure 6: A functional model for GCaMP molecular dynamics. A functional model for intramolecular interactions between cyclically permuted GFP (cpGFP; grey and green), calmodulin N (loops I and II; yellow) and C (loops III and IV;dark yellow)-lobes and RS20 (red) domains interacting with calcium ions (blue). High affinity for Ca2+is indicated by deeper sockets in the N- and C-lobes. Figure 6: A functional model for GCaMP molecular dynamics. A functional model for intramolecular interactions between cyclically permuted GFP (cpGFP; grey and green), calmodulin N (loops I and II; yellow) and C (loops III and IV;dark yellow)-lobes and RS20 (red) domains interacting with calcium ions (blue). High affinity for Ca 2+ is indicated by deeper sockets in the N- and C-lobes. Full size image The submillisecond responses we observe suggest a second possible kinetic pathway, in which high calcium levels can drive rapid binding to the low-affinity state of the N-lobe, which then would be sufficient to drive the CaM–RS20 conformational shift and chromophore protection. In this ‘N-like’ mode, C-lobe binding to Ca 2+ is not required, as evidenced by the fact that elimination of loop III or IV Ca 2+ binding sites leaves a functional (albeit low-affinity) probe. Finally, after removal of calcium, off-responses are limited in part by dissociation of the CaM–RS20 interface domain followed by Ca 2+ unbinding. A fruitful approach for future improvement would be to take advantage of high-throughput design methods, with which our approach is complementary. The mutations reported here can be integrated with recently reported high- R f variants [7] . The residues altered for high response and high per-molecule fluorescence reside in different probe domains [7] , opening the possibility of combinatorial approaches for continued improvement of performance. Another possibility that does not require further design improvements is to co-express multiple variants of differing affinities. Coexpression can expand detection range [35] . Such a combination of GECIs would give performance that had lower apparent cooperativity than any single GECI. Fast-GCaMP variant synthesis Point mutations to GCaMP3 were generated using the QuikChange II Site-Directed Mutagenesis Kit and Primer Design Program (Agilent Technologies). Coding regions were PCR amplified to attach restriction enzyme site linkers and cloned into the Not I and Xba I sites of the pET28b (Novagen) expression vector without removing the N terminus hexahistidine tag. BL21(DE3) E. coli (New England Biolabs, Ipswich, MA, USA) was transformed and starter cultures were grown in 10 ml LB medium supplemented with 50 mg l −1 kanamycin shaken at 225 r.p.m. at 37 °C. After 4 hours, each starter culture was added to 1 l of LB medium and maintained to OD=1.0 at 600 nm, the temperature reduced to 25 °C, and protein expression induced with 1 mM IPTG for 12–16 h. Cells were collected by centrifugation at 4500, r.p.m. at 4 °C and resuspended in anti-serine-protease wash buffer (25 mM Tris-Cl, 500 mM NaCl, 20 mM imidazole, 1 mM phenylmethylsulfonyl fluoride, pH 8.0) and lysed by two passes through the Emulsiflex C3 homogenizer (Avestin, Ottawa, ON, Canada). Cell debris were removed by 40 000 g centrifugation for 1 h at 4 °C. Clear lysates were purified by loading onto nickel-nitrilotriacetic acid Superflow resin columns (Qiagen) followed by 40 ml wash buffer. Protein was eluted with 500 mM imidazole and concentrated with 10 kDa Amicon Ultra centrifugal filters (Millipore), passed through a PD-10 desalting column (GE Healthcare), and resuspended in storage buffer (30 mM MOPS, 100 mM KCl, pH 7.20). Protein aliquots were frozen in ethanol chilled with dry ice and stored at −80 °C. Measurements on purified protein To measure the properties of purified Fast-GCaMP proteins, the Ca 2+ buffer used was 10 mM complexometry grade EGTA (Sigma-Aldrich) for steady-state measurements and 2 mM BAPTA (Molecular Probes) for kinetic measurements. Various free Ca 2+ concentrations were generated by mixing of high-Ca 2+ (Ca 2+ plus EGTA or BAPTA) and zero-Ca 2+ (EGTA or BAPTA alone) solutions [36] obtained from a commercial source (Invitrogen, Grand Island, NY) or made according to the method of Neher [42] . Free Ca 2+ concentrations were verified through titration of Fura-2 and Fura-4F (Molecular Probes). Free Ca 2+ concentrations were calculated using MaxChelator (C. Patton, maxchelator.stanford.edu ) assuming an ionic strength of 0.15 N for 10 mM K 2 H 2 EGTA, 100 mM KCl and 30 mM KMOPS (pH 7.20). Excitation and emission spectra were measured on a FluoroLog 3 spectrofluorometer (Horiba Jobin Yvon Inc., Edison, NJ, USA). For calcium-dependence, steady-state measurements were made using an F-2500 fluorescence spectrophotometer (488 nm excitation, 509 nm emission) running FL Solutions version 4.1 software (Hitachi, Japan) at 23 °C using 0.5–2 μM of purified protein suspended in either zero-Ca 2+ buffer or high-Ca 2+ buffer, followed by reciprocal dilution with the other buffer to reach free Ca 2+ concentrations between 0.01 and 10 μM. Calcium/magnesium selectivity was measured by competition assay in which 0.01–100 mM MgCl 2 was added to a solution containing 0.16–0.27 μM free Ca 2+ . Extinction coefficients ( ε 490nm ) were estimated using the absorption coefficient A 490nm at saturating [Ca 2+ ] free =39 μM. A 490nm is largely suppressed under conditions of low calcium and is eliminated by protein denaturation. Molar protein concentration was determined by measuring absorbance at 280 nm ( A 280nm ); in the cases listed in Table 1 , concentrations were further confirmed using A 447nm after alkali denaturation with 0.1 M NaOH for 3 minutes to eliminate fluorescence and generate an absorption band with ε 447nm =44 000 M −1 cm −1 (ref. 38 ). Quantum yield (QY) was determined by scaling F max /ε 490nm proportionally using QY=0.65 for GCaMP3 (ref. 7 ) as a benchmark. Stopped-flow measurements were performed at 25 °C or 37 °C with the AutoSF-120 and Stopflow version 1.0.1830 data acquisition software (KinTek, Austin, TX) using 488 nm xenon arclamp monochromator excitation and 525/40 nm filter (Chroma Technologies, Brattleboro, VT, USA) emission. The mixing dead time was <1 ms. Each shot consisted of 20 μl of reactant from each chamber. At least five shots were averaged and analyzed for 1–2 exponential components. Traces were fitted to a double exponential f ( t )= A 0 + A 1 exp(− k 1 t )+A 2 exp(− k 2 t ). To estimate the decay half-life ( t 1/2 ), f (0) was used in compensating for the instrument dead time and A 0 was used as the equilibrium fluorescence intensity. Imaging in Drosophila Fast-GCaMP variants (Fast-GCaMP-EF05, -RS06, -RS08 and -EF15) were cloned into the pJFRC-MUH (Addgene) plasmid containing 20 × UAS (GAL4 DNA binding domains). The transgene was inserted into the genome via PhiC31 integration (Rainbow Transgenic Flies, Inc., Camarillo, CA) into the attP2 landing of D. melanogaster . GCaMP5G was inserted into the attP40 landing site, which, when compared with the attP2 site, does not show differences in expression pattern/level [37] . Injected flies were crossed to a w 1118 strain and the significant transformants were identified. The Fru P1 Gal4 driver [38] was used to express GCaMP3, GCaMP5G, and all variants. Within the antennal nerve, therefore, both Fru+ olfactory and mechanosensory (JO) neurons expressed GCaMP; however, only JO neurons should respond to auditory stimuli. 20 × UAS-GCaMP3 also in attP2 was used as an expression-level-matched control [37] . Optical recordings were collected from 2-day-old virgin females. Flies were mounted ventral side up, with the dorsal side of the head, including antennae, protruding from the bottom surface of the platform [23] . The antennal nerve was imaged via dissection through the proboscis. To reduce motion, some muscles surrounding the brain were removed. Antennal nerve axons were imaged on a Zeiss LSM 710 two-photon laser scanning microscope at 15–16 frames per second using a 20 × water immersion objective (NA=1.0) at 256 × 256 resolution using pulsed 920 nm excitation (Coherent) and for detection, GaAsP photomultiplier tubes (Hamamatsu, Hamamatsu City, Japan) with 500–550 nm emission filters (Chroma Technologies, Brattleboro, VT). Laser intensity was maintained at <14 mW. Two types of sound stimuli were delivered via a calibrated sound delivery system [29] : 10 seconds of wild-type fly song and synthetic song pulse trains of 10–20 pulses separated by IPIs of 240, 120, 60 or 30 ms. Stimulus trials were separated by at least 20 s. Sound intensity (measured as particle velocity) reached 5.29 mm s −1 during natural song and 6.25 mm s −1 for synthetic song pulse trains. Peak Δ F / F 0 was calculated during the 5 s following stimulus onset. Decay phase t 1/2 was estimated through mono-exponential fitting for the first 5 s after termination of the song. ROIs were selected from a single imaging plane. Imaging of superior cervical ganglion neurons PRV expressing GCaMP variants were constructed by homologous recombination as previously described [39] . Proper fluorescent protein expression was assessed by epifluorescence microscopy. SCGNs were cultured from the lower mandible of embryonic rats [40] for 9–14 days. At 37 °C, SCGNs were either AM-loaded with 1–5 μM of fluorescent Ca 2+ indicator Oregon Green 488 BAPTA-1/AM (Life Technologies, Grand Island, NY) for 30 min or incubated for 60 min with 5 μl of viral stock (10 8 PFU ml −1 ) added to 3 ml of neurobasal media supplemented with B27, glutamine and nerve growth factor, followed by incubation in PRV-free media for 6–9 h. SCGNs were imaged at ~35 °C using a custom-built two-photon laser scanning microscope using pulsed 830 nm (OGB-1) or 920 nm (GCaMP) excitation from a Ti:sapphire laser (Mira 900, Coherent). Excitation power was kept at <15 mW at the backplane of the objective (× 40, NA 0.8 IR-Achroplan; Carl Zeiss, Thornwood, NY). Line scans (500 Hz) were made from neurites between 1 and 2 cell-diameters away from the soma. Data acquisition was controlled by ScanImage r3.6.1 (ref. 41 ). SCGNs were stimulated extracellularly by glass pipets filled with aCSF with tip diameters of ~5 μM placed ~0.5 cell-diameter away from the soma using 50-Hz pulse trains (1 ms, 5 V). Imaging of cortical L2/3 neurons L2/3 progenitor cells were transfected via in utero electroporation in timed-pregnant E-15 Swiss Webster mice (strain B6.129- Calb1tm1Mpin /J, The Jackson Laboratories, Bar Harbor, ME) with plasmids expressing GECIs under the CAGS promoter. At P14–21, 250 μM-thick cortical brain slices were prepared at in ice-cold artificial CSF (aCSF) containing (in mM) 126 NaCl, 3 KCl, 1 NaH 2 PO 4 , 20° D -glucose, 25 NaHCO 3 , 2 CaCl 2 and 1 MgCl 2 and saturated with 95% O 2 /5% CO 2 . Slices were preincubated at 34 °C for 40–60 min and then kept at room temperature. For recording, slices were transferred to an immersion-type recording chamber perfused at 2–4 ml min −1 with aCSF solution saturated with 95% O 2 /5% CO 2 at ~35 °C. L2/3 pyramidal neurons were shadowpatched with borosilicate patch recording electrodes (6–9 MΩ) filled with a solution containing (in mM, pH to 7.30 with KOH) 133 methanesulfonic acid, 7.4 KCl, 0.3 MgCl 2 , 3 Na 2 ATP and 0.3 Na 3 GTP, 290 mOsm. Electrophysiological signals were acquired with an Axopatch 200B amplifier and Clampex 8.0 software (Axon Instruments, Foster City, CA, USA). After whole-cell break-in, cells were held in current clamp mode (holding currents at −65 mV were −50 to −400 pA) and series resistances were 15–30 MΩ. Series resistance was monitored periodically and compensated by balancing the bridge. Spiking was induced through injection of current pulses at various amplitudes and durations and individual trials were separated by at least 10 s. L2/3 neurons were imaged using a custom-built two-photon laser scanning microscope using pulsed 830 nm (OGB-1) or 920 nm (GCaMP) excitation from a Ti:sapphire laser (Mira 900, Coherent). Excitation power was kept below 15 mW at the backplane of the objective (× 40, NA 0.8 IR-Achroplan; Carl Zeiss, Thornwood, NY). Line scans (500 Hz) were made from dendrites at least 1 cell-diameter away from the soma. Data acquisition was controlled by ScanImage r3.6.1 (ref. 41 ). How to cite this article: Sun, X. R. et al . Fast GCaMPs for improved tracking of neuronal activity. Nat. Commun. 4:2170 doi: 10.1038/ncomms3170 (2013).